Generation of organized germ layers from a single mouse embryonic stem cell Mammalian inner cell mass cells undergo lineage-specific differentiation into germ layers of endoderm, mesoderm and ectoderm during gastrulation. It has been a long-standing challenge in developmental biology to replicate these organized germ layer patterns in culture. Here we present a method of generating organized germ layers from a single mouse embryonic stem cell cultured in a soft fibrin matrix. Spatial organization of germ layers is regulated by cortical tension of the colony, matrix dimensionality and softness, and cell–cell adhesion. Remarkably, anchorage of the embryoid colony from the 3D matrix to collagen-1-coated 2D substrates of ~1 kPa results in self-organization of all three germ layers: ectoderm on the outside layer, mesoderm in the middle and endoderm at the centre of the colony, reminiscent of generalized gastrulating chordate embryos. These results suggest that mechanical forces via cell–matrix and cell–cell interactions are crucial in spatial organization of germ layers during mammalian gastrulation. This new in vitro method could be used to gain insights on the mechanisms responsible for the regulation of germ layer formation. Appropriate organization of three germ layers—endoderm, mesoderm and ectoderm—during gastrulation is essential for a developing embryo. Mechanistic studies on the morphogenesis of embryos in Drosophila, Caenorhabditis elegans , zebrafish and Xenopus have suggested important roles of mechanical forces in embryonic organization [1] , [2] , [3] , [4] , [5] . However, whether these embryos are similar to or different from those mammalian embryos remains unclear, because the study of mammalian embryo organization remains challenging due to the inaccessibility of in vivo embryos and lack of appropriate in vitro models. Embryoid bodies (EBs), formed by aggregation of embryonic stem (ES) cells (derived from inner cell mass cells of the blastocyst) in suspension, are used as in vitro models of differentiation [6] , [7] , but it has not been possible to manipulate generation of organized germ layers in EBs. A recent report shows that mouse ES cell aggregates can be induced to form polarized rosettes in vitro , followed by luminogenesis, similar to a developing embryo in vivo [8] . However, evidence for in vitro self-organization of three germ layers with correct positioning is still lacking. Here we present a novel method of generating embryoid colonies with organized germ layers from a single ES cell and show the factors controlling the germ layer organization. The endoderm, mesoderm and ectoderm layers are positioned at the inner, middle and outer layer of the growing colony, reminiscent of the layering of a generalized chordate gastrulating embryo. The layering of tissues as they express gastrulation markers can be inverted depending upon culture conditions. Generation of organized germ layers To dynamically monitor the status of pluripotency or mesodermal lineage differentiation of a single cell, we developed a mouse ES cell line (namely OGTR1) that stably expresses green fluorescent protein (GFP) driven by the Oct4 ( Pou5f1 ) promoter and red fluorescent protein (DsRed) driven by the Brachyury ( T ) promoter. To provide an appropriate mechanical and chemical niche to an ES cell, we plated the single OGTR1 ES cell within a soft fibrin gel [9] of 90-Pa ( Fig. 1a ), which is ~4-fold softer than the mouse ES cell [10] . In the presence of the self-renewal factor—Leukaemia Inhibitory Factor (LIF) [11] —the ES cell grew into a large round colony of >1,000 cells within 5 days at a doubling rate of ~11 h (ref. 10 ). The colony expressed a high level of Oct4 and no Brachyury, suggesting that these cells maintained pluripotency and self-renewing capacity ( Fig. 1a ; Supplementary Fig. 1 ). Interestingly, we did not observe heterogeneous expression of DsRed driven by the Brachyury promoter [12] . This observation was validated by RT–PCR ( Supplementary Fig. 2 ), consistent with previously published results [13] . In contrast, when plated in the absence of LIF for 5 days, a single OGTR1 ES cell divided and started to differentiate after ~48 h ( Supplementary Fig. 1 ), and grew into a colony of three distinct layers: a Gata6-positive layer indicative of endoderm at the inner layer, a Sox1-positive layer indicative of ectoderm at the middle layer and a DsRed (Brachyury)-positive layer indicative of mesoderm at the outer layer ( Fig. 1b,c ). The differentiation of the ES cells without LIF in the matrix was confirmed by RT–PCR as the expression of other lineage-specific genes was quantified ( Supplementary Fig. 2 ). Real-time qRT–PCR analysis of position-specific germ layer markers further verified that the observed ectoderm ( Fgf5 , Otx2 , Sox1 and Pax6 ), mesoderm ( Hand1 , Brachyury , Twist2 , FoxA2 and Mixl1 ) and endoderm ( Gata4 , Gata6 and Sox17 ) are truly bona fide ( Figs 2 , 3 , 4 ; Supplementary Fig. 3 ). In comparison, using a conventional hanging drop assay to generate EBs, ES cells failed to form distinct patterns of germ layers ( Supplementary Fig. 4 ), consistent with published results [6] , [7] , [14] . Plating a single ES cell on top of a 2D fibrin gel of 90-Pa resulted in both Gata6- and Sox1-positive layers appearing throughout the depth of the colony ( Supplementary Fig. 5 ), suggesting that a single ES cell plated in a very soft 3D niche grew more efficiently into self-organized germ layers than ES cells plated on a 2D substrate of the same softness. To assess the roles of cell–cell and cell–matrix interactions in germ layer organization, we disrupted cell–matrix interaction and cell–cell interaction. Blocking cell–fibrin interactions with the α v β 3 antagonist resulted in a dose-dependent appearance of the Gata6-positive layer at the outer layer, with little change to the position of either the Brachyury- or Sox1-positive layer ( Fig. 1d ; Supplementary Fig. 6 ), suggesting that engaging fibrin via α v β 3 integrin and the subsequent tension generation ( Fig. 6 ) may be important for the correct positioning of the endoderm layer. Blocking inter-E-cadherin adhesion with anti-E-cadherin antibodies ( Fig. 1e ) or addition of EGTA to disrupt calcium-sensitive, cadherin-mediated cell–cell adhesion ( Supplementary Fig. 7 ) completely abrogated the organization of the germ layers, consistent with reports that cell–cell interactions are crucial in early embryogenesis [15] , [16] , [17] , [18] , [19] , [20] , [21] , [22] . Although the underlying molecular mechanism for controlling the organization of each germ layer remains unknown (see our discussion below), these results are consistent with a recent finding that cell–cell interaction is important in stem cell differentiation [23] and myosin-IIA-mediated tension in the growing mouse embryoid colony is important in the appropriate positioning and organization of germ layers [22] . 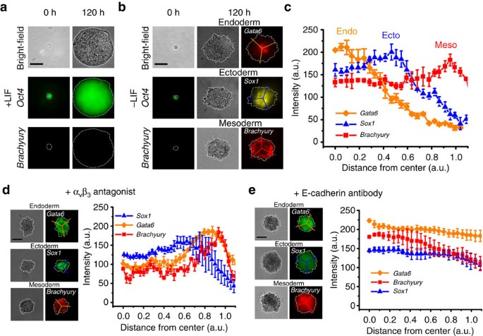Figure 1: Soft fibrin gels promote organization of germ layers. (a) Representative bright-field (top) and fluorescence (middle and bottom) images of a single ESC cultured in soft 3D fibrin gels in the presence of LIF (0 h) that formed a round spherical colony in 5 days (120 h). Strong EGFP fluorescence was observed (middle, ‘Oct4’), whereas no DsRed fluorescence was observed (bottom, ‘Brachyury’). (b) Representative images of a single ESC cultured in soft fibrin gels without LIF (0 h, the bright-field image is on the top and the fluorescence images on the middle and bottom, left column) that formed a colony with organized germ layers in 5 days (middle and left columns). Middle: bright-field images of colonies grown from three single cells; right: the presence of endo- and ectodermal cells was detected by immunofluorescence microscopy using anti-Gata6 and Sox1 antibodies, respectively, whereas DsRed fluorescence indicated the differentiation of mesodermal cells (Brachyury). Lines were used to acquire the fluorescence intensity data shown in (c). (c) Quantification of germ layer organization along with 0 (at the centre core) and 1 (at the colony boundary) arbitrary unit (a.u.) based on lines drawn on the fluorescence images on the left in (b). Mean±s.e.m. (d) Representative bright field (left) and fluorescence (middle) images and quantification of different germ layer markers (Sox1, Gata6 and Brachyury) 5 days after αvβ3 antagonist treatment (right). Single ES cells were treated with 20 μg ml−1of αvβ3 antagonist for 5 days in −LIF medium. Note that the endoderm layer was located at the outer periphery of the colony. Mean±s.e.m. (e) Representative bright-field (left) and fluorescence (middle) images in –LIF condition 5 days after anti-E-cadherin antibody (2 μg ml−1final concentration) treatment to block E-cadherin–E-cadherin adhesion. Germ layer organization was completely blocked. Quantification of different germ layer markers is shown on the right. Mean±s.e.m.; similar biological replicates of immunofluorescence staining were obtained from at least three independent experiments for each subfigure. W4 cells were used in all figures except foraand the mesoderm layer inbwhere OGTR1 cells were used. Scale bars, 50 μm. Figure 1: Soft fibrin gels promote organization of germ layers. ( a ) Representative bright-field (top) and fluorescence (middle and bottom) images of a single ESC cultured in soft 3D fibrin gels in the presence of LIF (0 h) that formed a round spherical colony in 5 days (120 h). Strong EGFP fluorescence was observed (middle, ‘Oct4’), whereas no DsRed fluorescence was observed (bottom, ‘Brachyury’). ( b ) Representative images of a single ESC cultured in soft fibrin gels without LIF (0 h, the bright-field image is on the top and the fluorescence images on the middle and bottom, left column) that formed a colony with organized germ layers in 5 days (middle and left columns). Middle: bright-field images of colonies grown from three single cells; right: the presence of endo- and ectodermal cells was detected by immunofluorescence microscopy using anti-Gata6 and Sox1 antibodies, respectively, whereas DsRed fluorescence indicated the differentiation of mesodermal cells (Brachyury). Lines were used to acquire the fluorescence intensity data shown in ( c ). ( c ) Quantification of germ layer organization along with 0 (at the centre core) and 1 (at the colony boundary) arbitrary unit (a.u.) based on lines drawn on the fluorescence images on the left in ( b ). Mean±s.e.m. ( d ) Representative bright field (left) and fluorescence (middle) images and quantification of different germ layer markers (Sox1, Gata6 and Brachyury) 5 days after αvβ3 antagonist treatment (right). Single ES cells were treated with 20 μg ml −1 of αvβ3 antagonist for 5 days in −LIF medium. Note that the endoderm layer was located at the outer periphery of the colony. Mean±s.e.m. ( e ) Representative bright-field (left) and fluorescence (middle) images in –LIF condition 5 days after anti-E-cadherin antibody (2 μg ml −1 final concentration) treatment to block E-cadherin–E-cadherin adhesion. Germ layer organization was completely blocked. Quantification of different germ layer markers is shown on the right. Mean±s.e.m. ; similar biological replicates of immunofluorescence staining were obtained from at least three independent experiments for each subfigure. W4 cells were used in all figures except for a and the mesoderm layer in b where OGTR1 cells were used. Scale bars, 50 μm. 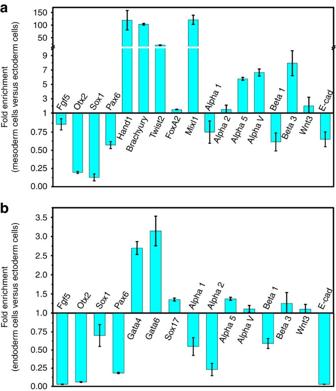Figure 2: Real-time qRT–PCR of different germ layers. Differentiated colonies from soft fibrin gels were extracted and cells of each germ layer were isolated using FACS sorting. (a) Mesoderm cells are compared with ectoderm cells. Expression of mesoderm markers:Hand1,Brachyury,Twist2,FoxA2andMixl1were higher (P<0.007,P<0.002,P<0.003,P<0.026 andP<0.012). Ectoderm markers such asFgf5,Otx2,Sox1andPax6were significantly lower (P<0.041,P<0.001,P<0.003 andP<0.012). Mesoderm cells express high levels of α5, αv, and β3integrin (P<0.002,P<0.008 andP<0.039). No significant difference was observed for α2integrin (P=0.31) and Wnt3 expression (P=0.62). Mean±s.e.m.n=3 independent experiments. (b) Endoderm cells are compared with ectoderm cells. Endoderm markers such asGata4,Gata6andSox17were highly expressed (P<0.010,P<0.031 andP<0.003), whereas ectoderm markersFgf5,Otx2,Sox1andPax6 were significantly lower (P<0.001,P<0.001,P<0.044 andP<0.001). Endoderm cells express high levels of α5integrin (P<0.008). No significant difference was observed for αvintegrin (P=0.21), β3integrin (P=0.38) and Wnt3 expression (P=0.19). These data suggest that ectoderm cells not only express high levels of α1β1integrin but also high levels of E-cadherin. Mean±s.e.m.;n=3 independent experiments. Full size image Figure 2: Real-time qRT–PCR of different germ layers. Differentiated colonies from soft fibrin gels were extracted and cells of each germ layer were isolated using FACS sorting. ( a ) Mesoderm cells are compared with ectoderm cells. Expression of mesoderm markers: Hand1 , Brachyury , Twist2 , FoxA2 and Mixl1 were higher ( P <0.007, P <0.002, P <0.003, P <0.026 and P <0.012). Ectoderm markers such as Fgf5 , Otx2 , Sox1 and Pax6 were significantly lower ( P <0.041, P <0.001, P <0.003 and P <0.012). Mesoderm cells express high levels of α 5 , α v , and β 3 integrin ( P <0.002, P <0.008 and P <0.039). No significant difference was observed for α 2 integrin ( P =0.31) and Wnt3 expression ( P =0.62). Mean±s.e.m. n =3 independent experiments. ( b ) Endoderm cells are compared with ectoderm cells. Endoderm markers such as Gata4 , Gata6 and Sox17 were highly expressed ( P <0.010, P <0.031 and P <0.003), whereas ectoderm markers Fgf5 , Otx2 , Sox1 and Pa x6 were significantly lower ( P <0.001, P <0.001, P <0.044 and P <0.001). Endoderm cells express high levels of α 5 integrin ( P <0.008). No significant difference was observed for α v integrin ( P =0.21), β 3 integrin ( P =0.38) and Wnt3 expression ( P =0.19). These data suggest that ectoderm cells not only express high levels of α 1 β 1 integrin but also high levels of E-cadherin. Mean±s.e.m. ; n =3 independent experiments. 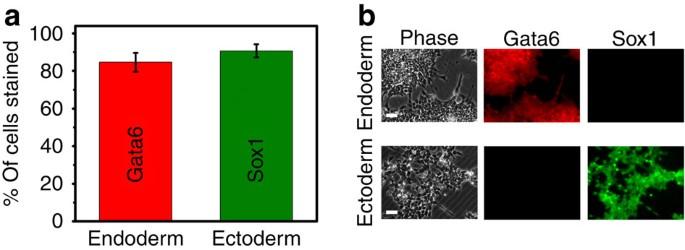Figure 3: Ectoderm and endoderm cells induced by exogenous chemical factors. (a) ESCs were differentiated with ActivinA (100 ng ml−1) or with retinoic acid (5 μM). Cells were then immunofluorescently labelled and the percentage of the stained cells was quantified using a haemocytometer. About 83% of the cells treated with ActivinA wereGata6–labelled, whereas ~90% of the cells treated with retinoic acid wereSox1-labelled;n=6 separate counts for each marker. (b) Representative phase contrast (left column), Gata6 (middle column) and Sox1 immunofluorescence images (right column) of endoderm (top row) and ectoderm (bottom row) cells. ESCs that were differentiated by ActivinA or by retinoic acid were each stained forSox1andGata6. ActivinA-treated cells are stained only byGata6(endoderm marker), whereas retinoic acid-treated cells are stained only bySox1(ectoderm marker). Real-time qRT–PCRs of these chemically differentiated cells are shown inFig. 4. Scale bars, 50 μm. Full size image Figure 3: Ectoderm and endoderm cells induced by exogenous chemical factors. ( a ) ESCs were differentiated with ActivinA (100 ng ml −1 ) or with retinoic acid (5 μM). Cells were then immunofluorescently labelled and the percentage of the stained cells was quantified using a haemocytometer. About 83% of the cells treated with ActivinA were Gata6 –labelled, whereas ~90% of the cells treated with retinoic acid were Sox1- labelled; n =6 separate counts for each marker. ( b ) Representative phase contrast (left column), Gata6 (middle column) and Sox1 immunofluorescence images (right column) of endoderm (top row) and ectoderm (bottom row) cells. ESCs that were differentiated by ActivinA or by retinoic acid were each stained for Sox1 and Gata6 . ActivinA-treated cells are stained only by Gata6 (endoderm marker), whereas retinoic acid-treated cells are stained only by Sox1 (ectoderm marker). Real-time qRT–PCRs of these chemically differentiated cells are shown in Fig. 4 . Scale bars, 50 μm. 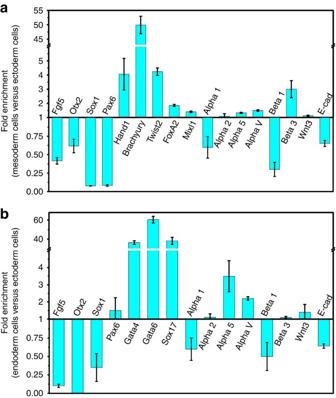Figure 4: Real-time qRT–PCR of different germ layers induced by exogenous chemical factors. Chemically differentiated ectoderm and endoderm cells were analysed to verify whether they arebona fide. (a) Mesoderm cells are compared with ectoderm cells. Expression of mesoderm markers:Hand1,Brachyury,Twist2,FoxA2andMixl1were higher (P<0.04,P<0.004,P<0.006,P<0.007 andP<0.02). Ectoderm markers such asFgf5,Otx2,Sox1andPax6were significantly lower (P<0.006,P<0.03,P<0.001 andP<0.001). Mesoderm cells express high levels of α5, αv and β3integrin (P<0.015,P<0.008 andP<0.041). No significant difference was observed for α2integrin (P=0.61) and Wnt3 expression (P=0.35). Mean±s.e.m.n=3 independent experiments. (b) Endoderm cells are compared with ectoderm cells. Endoderm markers such asGata4,Gata6andSox17were highly expressed (P<0.003,P<0.004 andP<0.01), whereas ectoderm markersFgf5,Otx2andSox1were significantly lower (P<0.001,P<0.001 andP<0.001). Endoderm cells express high levels of α5and αvintegrin (P<0.047,P<0.002). No significant difference was observed forPax6(P=0.38), α2integrin (P=0.21), β3integrin (P=0.1) and Wnt3 expression (P=0.48). These verify that ectoderm cells express high levels of E-cadherin and α1β1collagen-1 binding integrin. Mean±s.e.m.;n=3 independent experiments. Full size image Figure 4: Real-time qRT–PCR of different germ layers induced by exogenous chemical factors. Chemically differentiated ectoderm and endoderm cells were analysed to verify whether they are bona fide . ( a ) Mesoderm cells are compared with ectoderm cells. Expression of mesoderm markers: Hand1 , Brachyury , Twist2 , FoxA2 and Mixl1 were higher ( P <0.04, P <0.004, P <0.006, P <0.007 and P <0.02). Ectoderm markers such as Fgf5 , Otx2 , Sox1 and Pax6 were significantly lower ( P <0.006, P <0.03, P <0.001 and P <0.001). Mesoderm cells express high levels of α5, αv and β 3 integrin ( P <0.015, P <0.008 and P <0.041). No significant difference was observed for α 2 integrin ( P =0.61) and Wnt3 expression ( P =0.35). Mean±s.e.m. n =3 independent experiments. ( b ) Endoderm cells are compared with ectoderm cells. Endoderm markers such as Gata4 , Gata6 and Sox17 were highly expressed ( P <0.003, P <0.004 and P <0.01), whereas ectoderm markers Fgf5 , Otx2 and Sox1 were significantly lower ( P <0.001, P <0.001 and P <0.001). Endoderm cells express high levels of α 5 and α v integrin ( P <0.047, P <0.002). No significant difference was observed for Pax6 ( P =0.38), α 2 integrin ( P =0.21), β 3 integrin ( P =0.1) and Wnt3 expression ( P =0.48). These verify that ectoderm cells express high levels of E-cadherin and α 1 β 1 collagen-1 binding integrin. Mean±s.e.m. ; n =3 independent experiments. Full size image Figure 6: Colony tension impacts germ layer organization. 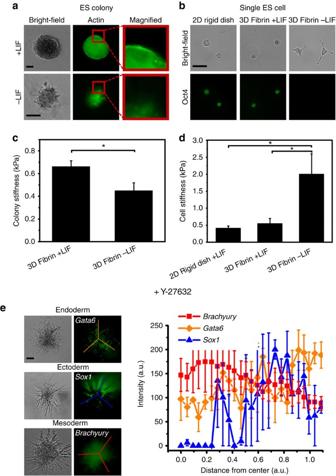Figure 6: Colony tension impacts germ layer organization. (a) Left: bright-field images of the colonies; middle: F-actin staining of the colony in the left; right: magnified areas of the boxes in the middle, showing much more F-actin in +LIF condition than in –LIF condition. (b) Representative bright-field (top) and fluorescence (bottom) images of individual cells (isolated from colonies maintained under conditions indicated on the top) on 2D rigid substrates. (c) Colony stiffness was measured after 5 days of culture for each isolated intact colony. Mean±−s.e.m.;n=84 for +LIF;n=80 for –LIF. (d) Individual cell stiffness. Individual cells were re-plated on 2D rigid substrate for 6 h before stiffness measurements were carried out. Mean±s.e.m.;n=28 for 2D rigid dish +LIF;n=53 for 3D fibrin +LIF;n=27 for 3D fibrin –LIF. (e) Representative bright field (left) and fluorescence (middle) images of the colonies treated with ROCK inhibitor Y27632 (25 μM) for 5 days (note that germ layers became disorganized and colonies exhibited extensive dendritic morphology); quantification of different germ layer markers is shown on the right. Mean±s.e.m. Similar results of immunofluorescence staining were obtained from at least three independent experiments for each subfigure. Scale bar, 50 μm. (*,P<0.023). OGTR1 cells were used in all subfigures except inaandewhere W4 cells were used. ( a ) Left: bright-field images of the colonies; middle: F-actin staining of the colony in the left; right: magnified areas of the boxes in the middle, showing much more F-actin in +LIF condition than in –LIF condition. ( b ) Representative bright-field (top) and fluorescence (bottom) images of individual cells (isolated from colonies maintained under conditions indicated on the top) on 2D rigid substrates. ( c ) Colony stiffness was measured after 5 days of culture for each isolated intact colony. Mean±−s.e.m. ; n =84 for +LIF; n =80 for –LIF. ( d ) Individual cell stiffness. Individual cells were re-plated on 2D rigid substrate for 6 h before stiffness measurements were carried out. Mean±s.e.m. ; n =28 for 2D rigid dish +LIF; n =53 for 3D fibrin +LIF; n =27 for 3D fibrin –LIF. ( e ) Representative bright field (left) and fluorescence (middle) images of the colonies treated with ROCK inhibitor Y27632 (25 μM) for 5 days (note that germ layers became disorganized and colonies exhibited extensive dendritic morphology); quantification of different germ layer markers is shown on the right. Mean±s.e.m. Similar results of immunofluorescence staining were obtained from at least three independent experiments for each subfigure. Scale bar, 50 μm. (*, P <0.023). OGTR1 cells were used in all subfigures except in a and e where W4 cells were used. Full size image Dependence of embryoid colony growth on matrix softness To further explore what dictates the growth rate of a single ES cell, we plated the cells within 3D fibrin matrices of varying softness. Five days after a single cell was plated, the resulting colony was much larger in the 90-Pa gel than the ones grown in the 420 or 1,050-Pa gel, in both the presence and absence of LIF ( Fig. 5a,b,e ). The proliferation rate of ES cells on 2D matrix was similar to those in 3D 90-Pa soft fibrin gels regardless of the 2D matrices stiffness, but the proliferation rate of cells in 3D fibrin gels decreased as matrix stiffness increased ( Supplementary Fig. 8 ), suggesting that a stiffer 3D matrix may pose a stronger physical barrier for the colony to increase its size as the cells divide. Interestingly, while colonies in all three matrices were spherical in the presence of LIF ( Fig. 5c ), the colonies in the 90-Pa matrix without LIF decreased their roundness much more significantly than those in 420 or 1,050-Pa matrix ( Fig. 5a(insets) ), suggesting that it is easier for the cells to move outward in the softest gel. The cells in the 90-Pa gel also increased DsRed expression slightly more than those in stiffer gels ( Fig. 5g ), whereas EGFP levels were similar ( Fig. 5d ). It is important to note that elevating the fibrin gel stiffness from 90 to 1,050 Pa was achieved by an increase in fibrin concentration from 1 to 8 mg ml −1 and thus a decrease in gel porosity. Hence it was difficult to discern whether it was the elasticity or the porosity of the gel that dictates the circularity of the colony. However, when a single ES cell was plated in the 3D fibrin gel of 90-Pa near the bottom of the plastic dish (~2 μm above it), it grew into a spread colony in the presence of LIF ( Supplementary Fig. 9 ). Since the porosity of the gel was the same for all cells in the gel, the cells near the bottom must have felt the stiffness of the rigid dish, consistent with the published reports [24] , [25] . 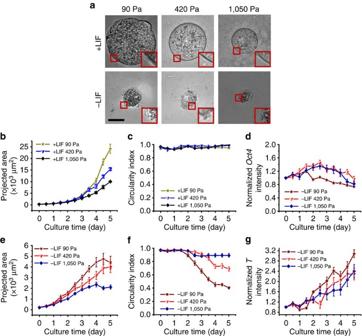These data suggest that it is the matrix stiffness, but not the matrix porosity, that dictates the spreading propensity of the ES cell. Figure 5: Matrix softness influences ES cell growth and differentiation. (a) Bright-field images of mESC colonies after 5 days of culture (grown from a single ESC) in 3D fibrin gels of different stiffness. Insets are magnified colony peripheries showing the surface roughness. Scale bar, 50 μm. (b) Summarized results of colony sizes in the presence of LIF (+LIF). (c) Circularity index in +LIF conditions. The circularity index is a measure of the roundedness of a colony. (d) Normalized EGFP intensity as a function of culture time in the absence of LIF (–LIF). (e) Projected areas as a function of culture time. (f) Circularity index in –LIF conditions. (g) Normalized DsRed intensity in –LIF conditions. Mean±s.e.m.;n=15 colonies for each condition inb–g. Data pooled from >3 independent experiments. OGTR1 cells were used to obtain the results of all figures. Figure 5: Matrix softness influences ES cell growth and differentiation. ( a ) Bright-field images of mESC colonies after 5 days of culture (grown from a single ESC) in 3D fibrin gels of different stiffness. Insets are magnified colony peripheries showing the surface roughness. Scale bar, 50 μm. ( b ) Summarized results of colony sizes in the presence of LIF (+LIF). ( c ) Circularity index in +LIF conditions. The circularity index is a measure of the roundedness of a colony. ( d ) Normalized EGFP intensity as a function of culture time in the absence of LIF (–LIF). ( e ) Projected areas as a function of culture time. ( f ) Circularity index in –LIF conditions. ( g ) Normalized DsRed intensity in –LIF conditions. Mean±s.e.m. ; n =15 colonies for each condition in b – g . Data pooled from >3 independent experiments. OGTR1 cells were used to obtain the results of all figures. Full size image Colony tension impacts germ layer organization To explore the potential role of tension in germ layer organization, we quantified stiffness of a whole-mouse ES cell colony isolated from the 3D fibrin gel matrix. Colonies cultured with LIF were stiffer than those without LIF ( Fig. 6c ), and colonies cultured with LIF had F-actins more concentrated at the periphery compared with those without LIF ( Fig. 6a ). In contrast, opposite to the whole colony’s mechanical property, single cells isolated from the colony were stiffer and more spread in the absence of LIF than those with LIF ( Fig. 6b,d ). This suggests that differentiation due to the absence of LIF stiffens single ES cells but not the whole colony, which was prevented from stiffening by the soft matrix. The stiffness of differentiated embryoid colonies at day 5 was similar to the values (~0.4 kPa) of embryonic discs [26] . Reduction of endogenous tension either with the addition of a Rho-associated kinase (ROCK) inhibitor or after addition of myosin-II inhibitor blebbistatin completely disrupted the proper organization of the germ layers, generating elongated cell protrusions with misaligned germ layers ( Fig. 6e ; Supplementary Fig. 10 ). siRNA knockdown of Myosin II-A and Myosin II-B also disrupted proper organization of germ layers ( Supplementary Fig. 11 ). In addition, downregulation of cellular tension with Blebistatin or with Y-27632 in +LIF conditions for 5 days resulted in loss of spherical morphology in the colonies but no differentiation or Brachyury-positive cells were observed ( Supplementary Fig. 12 ), suggesting that tension downregulation can influence colony morphology independent of differentiation by LIF. In contrast, when a constitutively active mutant of RhoA (RhoA-V14) [27] was transfected into the cells in +LIF condition, colonies remained spherical and pluripotent, whereas RhoA-V14-transfected colonies in the –LIF condition started to spread and positioned Brachyury-positive cells at the outer layer ( Supplementary Fig. 12 ). Taken together, these data suggest that the cytoskeletal tension in the actin filaments in the growing mouse embryoid colony may be important in the appropriate positioning and organization of the germ layers, consistent with published reports in lower animals [28] , [29] , [30] , [31] . Correct positioning of three germ layers At the very early developmental stage of mouse preimplantation embryos, the ball-shaped embryo grows and develops as it moves towards the uterus [32] , [33] . The cells of the epiblast begin to differentiate into three germ layers around embryonic-day 6 after its implantation into the uterine wall [34] , which consists mainly of type-1 collagen (collagen-1) [35] . We cultured single mouse ES cells in soft 3D fibrin gels in +LIF condition; then, we withdrew LIF after 11 h. At day 2.5 (after 60 h of culture in the 3D fibrin gel), the fibrin gels were gently dissolved. The intact individual colonies were isolated by mild centrifugation (56 g for 2 min) and transferred to the top of collagen-1-coated polyacrylamide (PA) gels of 1 kPa in –LIF conditions to mimic the signals during the implantation process ( Fig. 7a ). Remarkably, DsRed-positive cells formed a middle ring at day 5, two and a half days after adhesion on 2D collagen-1-coated substrates in –LIF conditions ( Figs 7b and 8 ; Supplementary Movie 2 ). Colonies transferred to 2D substrates of higher stiffness (3.5 or 8 kPa) gave rise to (non-spherical) spread colonies without a proper DsRed-positive layer ( Fig. 7b ). No in vivo data are available on the local stiffness of the endometrial epithelium when the embryo implants. However, in vitro data suggest that epithelial cells in general have a stiffness of ~1–5 kPa (ref. 36 ). Thus, our finding that a DsRed-positive layer formed in the middle of the colony after the colony was seeded on a 1-kPa substrate is consistent with the known stiffness range. Remarkably, immunostaining of colonies on 1-kPa gels showed a unique spherical morphology with self-organized germ layers reminiscent of generalized chordate gastrulae (ectoderm on the outside and endoderm at the inner most centre of the colony, with mesoderm in the middle) ( Figs 7c,d , 8 and 9 ; Supplementary Movies 1–3 ). In sharp contrast, colonies that were kept in the 3D fibrin matrix throughout the 5-day period ( Fig. 1b,c ) exhibited flipped mesoderm and ectoderm layers at day 5: endoderm at the inside, ectoderm in the middle and mesoderm at the outside. Interaction of the colony with collagen-1 (α 1 /α 2 β 1 integrins engage collagen-1; ref. 37 ) was found to be necessary for the formation of the proper germ layer organization as the transfer from 3D matrices to 2D surfaces with adhesion on other extracellular matrix proteins such as fibronectin (which engage α 5 β 1 and α v β 3 integrins [38] ) did not yield distinct organization of all three germ layers ( Supplementary Fig. 13 ). Consistent with the notion that normal morphogenesis of the inner cell mass is dependent on β 1 integrin [39] , [40] , but not on β 3 integrin [41] , [42] , our results indicate that only α 1 β 1 and/or α 2 β 1 integrins give rise to proper germ layer organization in our in vitro system. Reduction in colony attachment to collagen-1 resulted in no germ layer organization when the colonies were incubated in a medium containing anti-collagen 1 antibodies during transfer ( Supplementary Fig. 14 ), supporting the notion that the colony attachment to collagen-1 is specific. Studies have shown that the adherence of embryos with intact trophoblasts is significantly lower on laminin or fibronectin surface as compared with on collagen-1 substrates [43] . Furthermore, collagen-1 and β 1 integrin are highly expressed in EBs under hanging drop cultures [44] . Although no distinct organization of three germ layers was observed when colonies were transferred onto fibronectin-coated substrates, segregation of different cell types was observed ( Supplementary Fig. 13 ), consistent with the notion that fibronectin is necessary for the directed migration of mesodermal cells [45] . Taken together, these results indicate that local matrix dimensionality and colony–matrix interaction are critical to the proper organization of three germ layers, extending previous findings in lower animals that cell–cell tension plays important roles [15] . At present, the efficiency of generating each germ layer varied with this method. Proper organization of endoderm and mesoderm layers was simultaneously generated at relatively high efficiency (~50%, that is, ~50 out of every 100 transferred colonies had both layers in the correct position) and ~5% of the colonies (~5 out of every 100 transferred colonies) were found to be Sox1-positive cells that formed a ring-like layer at the periphery. Therefore, the success rate of generating correct positioning for all three germ layers was ~2.5%. Further refinement of this approach is needed to increase the efficiency of proper ectoderm generation. 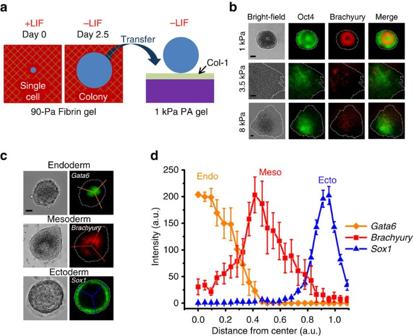Figure 7: Generation of three germ layer organization. (a) Schematic of the experimental protocol. A single OGTR1 ESC was grown in 3D 90-Pa fibrin gel in the presence of LIF (+LIF) for the first 11 h before switching to –LIF condition. At day 2.5, the individual colony is transferred to the top of collagen-1 (Col-1)-coated polyacrylamide gel (PA) of 1-kPa stiffness in the absence of LIF (−LIF). (b) Bright-field (left column) and fluorescence (second, third and right columns) images of ESC colonies maintained under conditions indicated on the left show positioning of a mesoderm layer (a DsRed-Brachyury expressing, donut-like ring) in the middle of the colony on top of Col-1-coated PA gels. Note that only on 1-kPa PA gels, the colony generated a mesodermal layer in the middle of the colony; spread colonies with randomly positioned mesodermal cells were found on stiffer substrates. EGFP is still expressed in the colony, suggesting that at this stage the colony is in transition between pluripotency and multipotency. (c) Representative bright-field (left) and fluorescence (right) images of colonies at day 5, after being transferred from 3D fibrin to 2D collagen-1 PA as described in (a). Endo- and ectodermal cells were stained by immunofluorescence microscopy using anti-Gata6 and Sox1 antibodies, respectively, whereas DsRed fluorescence indicated the differentiation of mesodermal cells (Brachyury). Lines were used to acquire the fluorescence intensity data shown in (d). (d) Quantification of germ cell organization as described inFig. 1c. Self-organized germ layers were properly replicated with endoderm at the core, mesoderm in the middle and ectoderm at the periphery. Mean±s.e.m.; at least three independent experiments showing similar results. Scale bar, 50 μm. The efficiency of Gata6-positive (endoderm) cells exclusively in the inner layer and the efficiency of Brachyury-positive (mesoderm) cells exclusively in the middle layer of the embryoid colony are ~50% (50 out of every 100 transferred colonies; >500 colonies quantified). The efficiency of Sox1-positive (ectoderm) cells exclusively in the outer layer of the embryoid colony is ~5% (5 out of every 100 colonies; >300 colonies were quantified). The efficiency of generating all three germ layers in the correct positioning is 2.6±0.28% (mean±s.e.m.; from nine separate experiments). In contrast, no proper positioning of any type of germ layer cells was found (0 out of 1,000 colonies) in the embryoid colonies when they were transferred to fibronectin-coated 2D PA substrates of 1 kPa (Supplementary Fig. 13). OGTR1 cells were used in all subfigures except the staining of endoderm and ectoderm in (c). Figure 7: Generation of three germ layer organization. ( a ) Schematic of the experimental protocol. A single OGTR1 ESC was grown in 3D 90-Pa fibrin gel in the presence of LIF (+LIF) for the first 11 h before switching to –LIF condition. At day 2.5, the individual colony is transferred to the top of collagen-1 (Col-1)-coated polyacrylamide gel (PA) of 1-kPa stiffness in the absence of LIF (−LIF). ( b ) Bright-field (left column) and fluorescence (second, third and right columns) images of ESC colonies maintained under conditions indicated on the left show positioning of a mesoderm layer (a DsRed-Brachyury expressing, donut-like ring) in the middle of the colony on top of Col-1-coated PA gels. Note that only on 1-kPa PA gels, the colony generated a mesodermal layer in the middle of the colony; spread colonies with randomly positioned mesodermal cells were found on stiffer substrates. EGFP is still expressed in the colony, suggesting that at this stage the colony is in transition between pluripotency and multipotency. ( c ) Representative bright-field (left) and fluorescence (right) images of colonies at day 5, after being transferred from 3D fibrin to 2D collagen-1 PA as described in ( a ). Endo- and ectodermal cells were stained by immunofluorescence microscopy using anti-Gata6 and Sox1 antibodies, respectively, whereas DsRed fluorescence indicated the differentiation of mesodermal cells (Brachyury). Lines were used to acquire the fluorescence intensity data shown in ( d ). ( d ) Quantification of germ cell organization as described in Fig. 1c . Self-organized germ layers were properly replicated with endoderm at the core, mesoderm in the middle and ectoderm at the periphery. Mean±s.e.m. ; at least three independent experiments showing similar results. Scale bar, 50 μm. The efficiency of Gata6-positive (endoderm) cells exclusively in the inner layer and the efficiency of Brachyury-positive (mesoderm) cells exclusively in the middle layer of the embryoid colony are ~50% (50 out of every 100 transferred colonies; >500 colonies quantified). The efficiency of Sox1-positive (ectoderm) cells exclusively in the outer layer of the embryoid colony is ~5% (5 out of every 100 colonies; >300 colonies were quantified). The efficiency of generating all three germ layers in the correct positioning is 2.6±0.28% (mean±s.e.m. ; from nine separate experiments). In contrast, no proper positioning of any type of germ layer cells was found (0 out of 1,000 colonies) in the embryoid colonies when they were transferred to fibronectin-coated 2D PA substrates of 1 kPa ( Supplementary Fig. 13 ). OGTR1 cells were used in all subfigures except the staining of endoderm and ectoderm in ( c ). 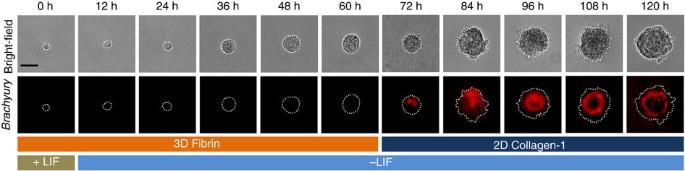Figure 8: Time course of formation of Brachyury-positive mesodermal middle layer. As described inFig. 7a, A single OGTR1 ESC was grown in 3D 90-Pa fibrin gel in +LIF condition for the first 11 h before switching to –LIF condition. After 60 h, the individual colony is transferred to the top of collagen-1-coated polyacrylamide gel in the absence of LIF. The Brachyury-positive cells were observed to localize or segregate at one end of the colony before sorting into a distinct middle mesodermal layer after 84 h. About 50% of the cells (out of 50 single ESCs) from >3 separate experiments that were tracked from time zero to 120 h showed similar results. Scale bar, 50 μm. Full size image Figure 8: Time course of formation of Brachyury-positive mesodermal middle layer. As described in Fig. 7a , A single OGTR1 ESC was grown in 3D 90-Pa fibrin gel in +LIF condition for the first 11 h before switching to –LIF condition. After 60 h, the individual colony is transferred to the top of collagen-1-coated polyacrylamide gel in the absence of LIF. The Brachyury-positive cells were observed to localize or segregate at one end of the colony before sorting into a distinct middle mesodermal layer after 84 h. About 50% of the cells (out of 50 single ESCs) from >3 separate experiments that were tracked from time zero to 120 h showed similar results. Scale bar, 50 μm. 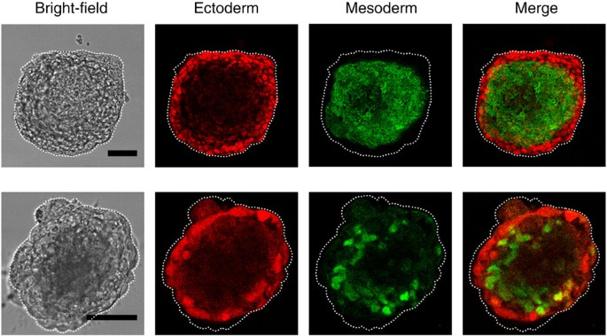Figure 9: Confocal images of ectoderm and mesoderm germ layers within the same colony. Representative images of two different colonies with bright field (left column), a distinct Pax6 ectoderm immunofluorescence at the outer layer (2nd column), a distinct Brachyury mesoderm immunofluorescence at the middle layer (3nd column) and merge fluorescence images (right column). Scale bar, 50 μm. From these staining data and those staining data of the colonies in the movies, assuming individual cells from each germ layer have the same volume, we estimate that endoderm, mesoderm and ectoderm layer cells are ~5%, 60% and 35% of the total cells, respectively. These results are representatives of >3 experimental replicates. Full size image Figure 9: Confocal images of ectoderm and mesoderm germ layers within the same colony. Representative images of two different colonies with bright field (left column), a distinct Pax6 ectoderm immunofluorescence at the outer layer (2nd column), a distinct Brachyury mesoderm immunofluorescence at the middle layer (3nd column) and merge fluorescence images (right column). Scale bar, 50 μm. From these staining data and those staining data of the colonies in the movies, assuming individual cells from each germ layer have the same volume, we estimate that endoderm, mesoderm and ectoderm layer cells are ~5%, 60% and 35% of the total cells, respectively. These results are representatives of >3 experimental replicates. Full size image Time course of the Brachyury gene expression shows that Brachyury-positive cells localize at one end of the embryoid colony before sorting into a middle mesodermal layer ( Fig. 8 ). When these embryoid colonies on 2D collagen-1 substrates were then encapsulated in 3D fibrin gels, the Brachyury-positive mesoderm cells distributed outwards to the outer layer ( Fig. 10b ). Conversely, late-stage embryoid colonies that formed the outer mesoderm layer in the 3D fibrin gels distributed toward the middle layer when they were transferred onto 2D collagen-1 substrates ( Fig. 10a ), suggesting that self-organization of embryoid colony is due to differential adhesion of cells from different germ layers since in the 3D fibrin gels the outer layer cells engage α v β 3 integrin, whereas on the 2D gels the outer layer cells engage α 1 β 1 integrins. Immunofluorescence staining of β 1 integrin ( Supplementary Fig. 15 ) and qRT–PCR results ( Figs 2 and 4 ) show that ectoderm cells expressed higher levels of α 1 β 1 integrin that preferentially binds to collagen-1 than the other two germ layer cells. These results suggest that differential integrin expression and engagement influence germ layer organization. 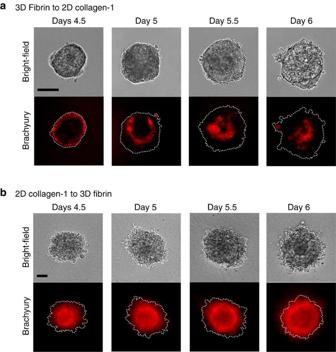Figure 10: Self-organization of the embryoid colony is due to differential adhesion of germ layer cells. (a) A single ESC was cultured in 3D soft fibrin gels in the absence of LIF. When Brachyury-positive cells were distinctly observed at the outer layer at 4.5 days, the gel was dissolved and colonies transferred to 2D collagen-1-coated PA gel. The Brachyury-positive outer layer was observed to move inwards to the middle layer by day 6. (b) As described inFig. 7a, ESCs were first cultured in 3D soft fibrin gels before being transferred to 2D collagen-1-coated PA gel after 60 h. At day 4.5 when Brachyury-positive cells were distinctly expressed at the middle layer, the colonies were encapsulated with 3D soft fibrin gel. The Brachyury-positive middle layer was observed to move outwards to the outer layer by day 6. These results suggest that the colony self-organizes on the basis of preferential binding of mesodermal cells to fibrin and ectodermal cells to collagen-1. Scale bar, 50 μm. These results are representative of >3 experimental replicates. Figure 10: Self-organization of the embryoid colony is due to differential adhesion of germ layer cells. ( a ) A single ESC was cultured in 3D soft fibrin gels in the absence of LIF. When Brachyury-positive cells were distinctly observed at the outer layer at 4.5 days, the gel was dissolved and colonies transferred to 2D collagen-1-coated PA gel. The Brachyury-positive outer layer was observed to move inwards to the middle layer by day 6. ( b ) As described in Fig. 7a , ESCs were first cultured in 3D soft fibrin gels before being transferred to 2D collagen-1-coated PA gel after 60 h. At day 4.5 when Brachyury-positive cells were distinctly expressed at the middle layer, the colonies were encapsulated with 3D soft fibrin gel. The Brachyury-positive middle layer was observed to move outwards to the outer layer by day 6. These results suggest that the colony self-organizes on the basis of preferential binding of mesodermal cells to fibrin and ectodermal cells to collagen-1. Scale bar, 50 μm. These results are representative of >3 experimental replicates. Full size image While colony–matrix interaction plays a role in germ layer positioning, stimulation of signalling pathways by soluble factors is well known to be important in differentiation and development of embryos. Wnt signalling components have been reported to be essential for the establishment of primitive streak and mesoderm formation [46] , [47] . In our EBs, expression of Wnt3a and Bmp4 were detected a day before Brachyury appearance and both were found to form similar polar ends before dispersing throughout the whole colony ( Supplementary Fig. 16 ). Since Wnt signalling mediates the anterior–posterior polarity and axis formation in EBs [14] , we explored the role of Wnt, Bmp4 and nodal in the organization of different germ layers. Without exogenous signals, cells cultured in 3D soft fibrin gels for 5 days formed mesoderm cells at the outer layer. However, low concentrations of Wnt3a, Bmp4 or ActivinA (which activates the nodal pathway [48] ) all resulted in formation of middle layer Brachyury-positive mesoderm cells ( Supplementary Fig. 17 ). Supplementing the medium with Dkk1 (a Wnt antagonist) caused the mesoderm cells to form the inner layer in the case of Wnt3a and ActivinA, but not Bmp4 ( Supplementary Fig. 17 ). Interestingly, Bmp antagonist Noggin along with the activation of Wnt, Bmp and nodal caused the cells with Brachyury expression to form the outer layer. Suppressing Bmp alone without the activation of other signals caused the cells to undergo apoptosis ( Supplementary Fig. 17 ). Together with the time course results of Brachyury expression ( Fig. 8 ), we conclude that Wnt signalling is essential in early formation of anterior–posterior polarity, and continuous activation or inhibition of Wnt, Bmp4 or nodal signals for 5 days gives rise to a shift in germ layer position ( Supplementary Fig. 17 ). The organization of germ layers observed at day 5 in this study is of a relatively late-stage in embryogenesis, after the establishment of primitive streak and anterior–posterior polarity [14] . Although we do not know at the present time the underlying mechanism for controlling the organization of the germ layers when the Wnt signalling pathway is modulated, together with our findings that colony tension impacts germ layer organization, differentiation-related processes and/or molecules in germ layer organization such as Wnt3, Bmp4 and nodal as well as tension may play crucial roles in the formation of organized germ layers. When ES cells were cultured in soft 3D fibrin gels under –LIF conditions throughout the first day of the culture (day 0) and transferred to 2D collagen-1-coated PA substrates at day 2.5, they did not maintain their spherical shape. Rather, the colony spread out and formed a monolayer of cells within a day of adhesion to the 2D substrate ( Supplementary Fig. 18 ). These results suggest that the timing of withdrawing the soluble self-renewal factor LIF as well as appropriate substrate stiffness, matrix dimensionality and colony–matrix mechanical tension are critical to the generation of self-organized germ layers in this in vitro embryo model. Taken together, our results show that the development of the OGTR1 mouse ES cell line and the culture of ESCs in soft 3D fibrin gels provide a useful platform for further studies on the formation of organized germ layers. The present study demonstrates that a spherical colony with proper germ layer arrangement of endoderm, mesoderm and ectoderm from the inner layer to the outer layer can be generated from a single mammalian ESC by controlling colony tension and anchorage-dependent cell–matrix interaction. A report of an in vitro assay reveals that the frequency of development of early mouse embryos on 1-kPa collagen-1 gels is greater than that on rigid substrates of 1 GPa (ref. 49 ), suggesting that our assay using collagen-1-coated 1-kPa gels might be useful and relevant. This method could provide an in vitro model for exploring mechanisms of tissue morphogenesis during mammalian germ layer formation. The outer and the inner layers of gastrulating mouse embryos at E6.5–8.0 differentiate into the visceral endoderm and the embryonic ectoderm, respectively [50] . With regard to the spatial organization of three germ layers, the embryoid colony is similar to the mouse embryo at E9.0 after a process of rotation that results in the endoderm locating at the inner layer and the ectoderm locating at the outer layer. However, the cells in the E9.0 mouse embryo are more specialized than those of the embryoid colony; mouse and human embryos at the gastrulation stage have the shapes of cylinders and plates, respectively, different from the spherical shape of the embryoid colony observed in the current study. Therefore, it will be interesting to see what cell types and shape the self-organized embryoid colony in long-term cultures (>5 days) will develop into. A recent report demonstrates that the engagement of β 1 -integrins with the extracellular matrix proteins enables self-organization of mouse ESCs to form polarized rosettes that initiate luminogenesis similar to days 2.5–5.0 embryos in vivo [8] . Consistently, our results demonstrate that interactions of the embryoid colony with collagen-1 are necessary for the formation of proper germ layer organization. In addition to the recent findings in the culture conditions that stimulate implantation and allow ES cells to develop into epiblast-like structures [8] , we demonstrate that the culture of ES cells can be taken further to establish distinct lineages using specific protocols. Our current approach shows the ability to generate self-organization of three germ layers in vitro , a stage later than the polarized rosettes. However, the detailed events and underlying mechanisms leading up to the organized germ layer patterns remain to be elucidated. Our finding that specific cell–matrix interaction and matrix dimensionality are crucial in germ layer positioning is further strengthened by the result that the mesoderm layer distribution is inverted (from the middle layer to the outer layer) when the colony is transferred from a 2D collagen-1 surface into a 3D fibrin gel ( Fig. 10 ). Our observation that blocking matrix (fibrin)–integrin interaction and thus potentially myosin-II-dependent tensile forces across the integrins results in the endoderm layer moving from the inner layer to the outer layer ( Fig. 1c,d ) suggests that the appropriate positioning of the endoderm layer depends on the tensile forces of the cells. On the other hand, the mesoderm layer locates from the outer layer ( Fig. 1c ) to the middle layer ( Fig. 7c,d ) when the embryoid colony is transferred from a 3D matrix substrate to a 2D matrix substrate, and the ectoderm layer moves in the opposite direction (compare Fig. 1c with Fig. 7d ), suggesting that asymmetric tensile force distribution and possibly magnitudes and directions of compressive forces may play critical roles in mesoderm/ectoderm layer organization, in addition to specific integrin subtypes (that is, collagen-1 versus fibronectin; see Fig. 7c and Supplementary Fig. 13 ). A recently developed novel oil-droplet force transducer system [51] might be used to elucidate these questions and to quantify magnitudes, direction and distribution of forces surrounding growing embryoid colonies, as increasing in vivo evidence suggests that contractile acto-myosin networks drive cell shape changes during morphogenesis [52] . The position-specific gene expression patterns from the cells isolated from the embryoid colonies in the 3D fibrin gels are in general consistent with and similar to those chemically induced (differentiation) gene patterns, but there are a few quantitative differences in a few genes (for example, Hand1 , Brachyury , Twist2 , Gata4 , Gata6 and Sox17 ). It will be interesting to determine what accounts for these quantitative differences. It has been shown that exogenous biophysical signals can be transmitted through the cytoskeleton and into the nucleus to dissociate protein–protein complexes in the Cajal bodies [53] ; however, at present the molecular mechanisms of how matrix rigidity and dimensionality influence the differentiation of ESCs and organization patterns of germ layers remain elusive. Published reports show that the Yes-associated protein (YAP) and TAZ are important in the matrix-rigidity-dependent differentiation of mesenchymal stem cells [54] and motor neuron differentiation of human pluripotent stem cells [55] . It will be interesting to see whether YAP/TAZ and/or other unknown factors play a role in early embryogenesis and germ layer organization. Creation of OGTR1 mESC cell line Unless otherwise noted, the restriction enzymes and DNA-modifying enzymes used in this study were obtained from New England Biolabs (Ipswich, MA, USA). pGTIV2 (ref. 56 ) was digested with ClaI and NsiI to remove an intervening sequence that contains one PvuII site, and ligated with a ClaI-NsiI linker (Invitrogen, Carlsbad, CA). This modified pGTIV2 was further digested with NotI and PvuII to obtain a cassette that contains Gtx motifs [57] , Venus [58] and polyadenylation signals (referred to as IVpA). The IVpA cassette was ligated into pBluescriptIIKS(−) sequentially digested with SalI and NotI. Before NotI digestion, the cohesive ends generated by SalI digestion were blunt-ended with the Klenow fragment (Invitrogen). The resulting vector was named pBS_IVpA. After a unique EcoRI site was introduced at an XbaI site in pBS_IVpA by a linker (Invitrogen), Venus in pBS_IVpA was removed by digestion with NcoI and EcoRI, and replaced with modified Venus that lacks a stop codon (TAA). This modification of Venus was carried out by PCR with Phusion DNA polymerase and the following primers: forward 5′-ATGATATCGCCACCATGGTGAGCA-3′; reverse 5′-TCGAATCTGTACAGCTCGTCC-3′ (ref. 59 ). The resulting pBS_IVpA with modified Venus was digested with EcoRI and XbaI to clone the puromycin-resistant gene ( Puro r ) with the self-cleaving peptide T2A [60] at the 5′ end of Puro r , which was obtained from pCAG_T2APuro [59] . The resulting vector, namely pBS_IV2AP, was digested with NotI and ClaI and subsequently ligated with self-annealed oligonucleotides that encode restriction enzyme sites of NotI, EcoRV, PmeI, AflII, PacI, NheI and HpaI (sense: 5′-GGCCGCGATATCGTTTAAACTTAAGTTAATTAAGCTAGCGTTAAC-3′; antisense 5′-CGGTTAACGCTAGCTTAATTAACTTAAGTTTAAACGATATCGC-3′; Integrated DNA Technologies (IDT), Coralville, IA, USA). This linker contains a NotI site at the 5′ end and a compatible but mutated ClaI site at the 3′ end. The resulting vector was designated pBS_MCSIV2AP. Then, Venus in pBS_MCSIV2AP was removed by digestion with NcoI and EcoRI and replaced with DsRedT3 (ref. 61 ) obtained from pCAG_DsRedT2AP (refs 59 , 62 ). The resulting vector was named pBS_MCSIR2AP. An XhoI site was introduced at the NotI site in pBS_MCSIR2AP by a linker (IDT). The resulting vector was designated pBS_MCSIR2APx. To build a drug resistance cassette, the PGK promoter and the blasticidin-resistant gene ( Bsd r ) were obtained from pGTLox4 (kindly provided by Dr William L. Stanford, University of Ottawa, Ottawa, Canada) that was digested with EcoRI and ScaI, and subcloned into EcoRI and SmaI-digested pBluescriptIIKS(−) that has polyadenylation signals cloned at the XbaI site. The resulting vector, namely pPGKBsrpA, was digested with XhoI and ligated with an XhoI-digested cassette obtained from pBS_MCSIR2APx that harbours multiple cloning sites, Gtx motifs, DsRedT3 linked with Puro r via T2A and polyadenylation signals. The final vector, referred to as pMCSIRPPB, has unique AflII, ApaI, HpaI, KpnI and NheI sites to clone a gene-specific promoter. The gene regulatory sequence of the T gene was amplified by PCR using a BAC (RP23-444I17, BACPAC Resources Center, Children’s Hospital Oakland Research Institute, CA, USA) as a template and the following primers: EcoRV-pT-F, 5′-AAGATATCTCCCTCTCAGGTGCGCGCAG-3′; NheI-pT-R, 5′-TTGCTAGCCTCCCGCCACCCTCTC-3′ (IDT). These primers were designed to amplify a genomic region between −529 and +152 relative to the transcriptional initiation site, which regulates T expression in the streak-derived mesoderm but not in the axial mesoderm [63] . The PCR product digested with EcoRV and NheI was cloned into pMCSIRPPB sequentially digested with KpnI and NheI. Before NheI digestion, cohesive ends of pMCSIRPPB generated by KpnI digestion were blunt-ended by T4 DNA polymerase. Cloned DNA sequence identity was verified by sequencing. The purified resulting vector, namely pTIRPPB, was transfected to mouse ES cells that express EGFP under the Oct3/4 promoter (OGR1) [12] , [59] , [62] , [64] , [65] by FuGene HD (Roche Applied Science, Indianapolis, IN, USA) essentially as previously described [59] . Blasticidin-resistant clones, namely OGTR1, were isolated and expanded for analysis. Stochastic expression of DsRedT3 was observed in OGTR1 cultured as undifferentiated [11] , [66] . mESC culture A wild-type mESC line (W4, 129S6/SvEvTac) was cultured and used as described [62] . These cells were further used to grow single individual cells into colonies and immunostained for endoderm, mesoderm or ectoderm germ layers. In addition, the OGTR1 mESC line described above was used in this study. These undifferentiated mESCs were cultured and maintained in the medium consisting of high glucose-Dulbecco’s Modified Eagles Medium (Invitrogen) supplemented with 15% ES-qualified fetal bovine serum (Invitrogen), 2 mM L-glutamine (Invitrogen), 1 mM sodium pyruvate, 0.1 mM nonessential amino acids (Invitrogen), 1% penicillin–streptomycin, 0.1 mM beta-mercaptoethanol (Sigma) and 1,000 U ml −1 recombinant LIF (ESGRO; Millipore) at 37°C in 5% CO 2 . Cells were passaged every 2–3 days at a ratio of 1:6 using TrypLE (Invitrogen). Culture medium was changed daily. Recombinant Wnt3a, Bmp4, ActivinA, Dkk1 and Noggin were obtained from R&D Systems. Cell and colony stiffness measurement Cell and colony stiffness were measured using magnetic twisting cytometry [9] , [62] , [67] . A ferromagnetic bead of ~4 μm in diameter is coated with Arg-Gly-Asp (RGD) peptides and bound to the apical surface of cells. Magnetic twisting cytometry allows us to control the loading frequency and the duration as well as the magnitude of force applied to the cell. The bead displacement amplitude can then be correlated to the applied mechanical force to determine the cell stiffness. Dissolving fibrin gels The 3D fibrin gels were dissolved using a solution mixture of Collagenase (Sigma C0130) and Dispase II (Sigma D4693) [68] . Collagenase and Dispase II were diluted by 2 ml PBS at the final concentration of 0.08 and 0.4% ( w / v ), respectively. Adding 400 μl of the solution to a well (24-well plate size) containing 250 μl fibrin gel with 600 μl of existing culture medium will take 30 min to dissolve at 37 °C. The colony shape changed little before and after transfer from 3D to 2D, suggesting that the Collagenase- and Dispase II-dissolving solution did not affect the colony integrity much. After centrifuging at 500 r.p.m. (~56 g) for 2 min, the colonies were re-suspended by pipetting a few times. About 80–100 colonies were pipetted and transferred to the centre of the dish where the PA gel was. 3D fibrin gel cell culture and differentiation assay Twenty-four-well plates were used to culture mESCs in the 3D fibrin gel. mESCs were first trypsinized using TrypLE (Invitrogen) and suspended in the complete ESC culture medium as described above. For each well, 500 ESCs were prepared in 125 μl of the medium. Cells in suspension were then placed on ice while the subsequent steps were executed. Salmon fibrinogen solid (Reagent Proteins) was dissolved in 125 μl of T7 buffer (pH 7.4, 50 mM Tris, 150 mM NaCl) to a concentration of 2 mg ml −1 . The cells in suspension were then added to the fibrinogen mixture at a ratio of 1:1, making the resulting fibrinogen concentration to 1 mg ml −1 . Five microlitres of thrombin (0.1 U μl −1 ) were then added to each well of the 24-well plate. A total of 250 μl of the cell–fibrinogen mixture was added to each well and mixed with thrombin (Reagent Proteins). The plate was then incubated at 37°C for 10 min to solidify before adding 1 ml of the complete ESC culture medium. Two-dimensional fibrin gels were prepared using the same protocol as 3D fibrin gels but without premixing of cells. After the gels were made, mESCs were seeded on top of the fibrin gels. Cells were cultured in 3D or 2D fibrin gels up to 5 days. For differentiation assays, ESCs were cultured in a medium without LIF (-LIF). The α v β 3 -blocking antagonist cRGDfV (Enzo Life Sciences) was pre-diluted in the normal culture medium to the indicated concentrations before being used for cell treatment. Apoptosis staining Propidium iodide (PI, Sigma) was used to label apoptotic ESCs. Colonies after 5 days of culture were labelled with PI according to the manufacturer’s protocol. Staining of PI indicates that none or only a few cells within the colonies are apoptotic ( Supplementary Fig. 19 ). EB formation assay Hanging drop cultures were prepared using 25 μl droplets, each having 600 cells to initiate EB formation [69] . Undifferentiated ESCs were trypsinized and allowed to form EBs in the bottom of the hanging drops made with the ES medium without LIF for 5 days. The different germ layers were detected by immunofluorescence microscopy. Immunofluorescence staining ESCs in 3D fibrin gel culture were fixed with the fix buffer consisting of 4% formaldehyde (BioLegend) for 20 min at room temperature. Cells were then permeabilized with 0.5% Triton X-100 (BioLegend) for 2 min and treated with blocking buffer made of 2% BSA in PBS for 1 h. To examine the presence of different germ layers, an anti-Gata6 primary antibody (Santa Cruz Biotechnology) was used to label endoderm; an anti-Brachyury primary antibody (Abcam) was used to label mesoderm; and an anti-Sox1 primary antibody (Abcam) was used to label ectoderm. Detection of germ layer types was performed using appropriate Alexa-conjugated secondary antibodies (Invitrogen). Cells were incubated with all primary antibodies (diluted with 2% BSA buffer at a ratio of 1:200) overnight at 4 °C. After being washed to remove unbound primary antibodies, cells were incubated with the secondary antibody for 4 h under dark conditions. For E-cadherin staining, permeabilized cells were incubated with a rabbit monoclonal anti-E-Cadherin antibody conjugated with Alexa-488 (Cell Signaling) for 1 h before examining under a fluorescence microscope. Negative immunofluorescence control experiments were performed by staining colonies that were cultured in +LIF condition for 5 days for endoderm, mesoderm and ectoderm layers ( Supplementary Fig. 20a ). The undifferentiated colonies were first treated with primary antibodies followed by the secondary antibody. For each germ layer, it was observed that there were small negligible areas within the colony that were stained. We therefore decided to stain colonies cultured in –LIF 3D conditions at day 5 with individual primary antibodies or individual secondary antibody ( Supplementary Fig. 20b ). Colonies treated with primary antibodies alone did not show any fluorescence, whereas colonies treated with secondary antibody alone had some small fluorescent spots. These suggest that there is some nonspecific staining of secondary antibody that has not been unwashed out. RNA interference Cells were transfected with siRNA using Lipofectamine 2000 (Invitrogen) according to manufacturer’s protocol. Mouse siRNA silencer for Myh9 gene Myosin II-A (NMHC II-A) (Invitrogen, no. 262920) and mouse siRNA silencer for Myh10 gene Myosin II-B (NMHC II-B) (Invitrogen, no. 176254) were obtained from Life Technologies. Silencer Negative Control No. 1 siRNA (Invitrogen, AM4611) was used as control. Circularity index The circularity of colonies was calculated using the formula of 4π × (area)/(perimeter) 2 . A perfect circle has a value of 1.0. Confocal imaging After colonies were fixed and immunofluorescently labelled, confocal microscopy was performed using a Leica SP8-STED microscope to obtain 3D reconstructive images of the colonies ( Supplementary Movies 1–3 ). A × 20 oil immersion objective was used. Each colony was imaged using 250 z -stack images with each step of ~0.8 μm. Fluorescence was detected using a photomultiplier tube or Hybrid Detector (HyD). RT–PCR analysis RNA of mESC spheroids from 3D fibrin gel culture was extracted using Trizol reagent according to the supplier’s instruction (Invitrogen). Extracted mRNA was then used for reverse transcription using SSIIRT (Invitrogen). The cDNA was then amplified using a PCR kit (QIAGEN). The expression of Nanog, Oct3/4, Sox2, Fgf5, Otx2, Sox1, Hand1, Brachyury, Twist2, Gata4, Gata6 and Sox17 mRNA was examined. The mRNA of glyceraldehyde-3-phosphate dehydrogenase (GAPDH) was used as an internal control. The primer sequences are shown in Supplementary Table 1 . Real-Time qRT–PCR analysis OGTR1 cells were cultured for 5 days in –LIF 3D soft fibrin gels for 5 days. Fibrin gels were dissolved and the differentiated colonies were dissociated with 0.25% TrypLE (Invitrogen), resuspended in PBS with 1% serum. Cells were isolated into DsRed::Brachyury fluorescence-expressing and DsRed-negative cells using fluorescence-activated cell sorting (FACS; Beckman). First we used chemical differentiation factors to analyse the DsRed-negative cells. The DsRed-negative cells were differentiated into endoderm-like cells with continuous treatment of 100 ng ml −1 of ActivinA [70] for 3 days in regular –LIF medium on gelatin-coated six-well plates. The DsRed-negative cells were differentiated into ectoderm-like cells by gradually reducing serum in –LIF medium till the second day where the medium was replaced with serum-free medium supplemented with 5 μM retinoic acid [71] for the remaining 24 h on gelatin-coated six-well plates; Fig. 3 ). After treatment with retinoic acid or with ActivinA, the DsRed-negative cells expressed high levels of E-cadherin or low levels of E-cadherin ( Fig. 4 ). To obtain position-specific gene information, we used the knowledge gained from the chemical differentiation method and isolated W4 cells (OGTR1 cells were not used to avoid florescence interference during cell sorting) that had been grown for 5 days in the soft fibrin gels in –LIF condition and then added them briefly to the top of the fibrin (binds to a v β 3 integrin) gels for 5 min. The attached cells are likely to be mostly mesoderm-like cells. We gently collected the unattached cells (presumably a mixture of ectoderm- and endoderm-like cells) in the medium and stained them using anti-E-cadherin antibodies (primary anti-E-cadherin antibody (rat) DECMA-1; secondary antibody anti-rat-IgG FITC; both from Sigma), and then we sorted these cells using FACS into high and low E-cadherin-expressing cells ( Supplementary Fig. 3 ). The sorted DsRed-positive cells (from the OGTR1 cell line), high E-cadherin expression cells and the remainder low E-cadherin expression cells were then analysed by real-time qRT–PCR ( Fig. 2 ). All cDNA sequences were retrieved from the National Center for Biotechnology Information (NCBI) database. All data were analysed using comparative cycle threshold method for relative gene expression against GAPDH. The primer sequences are shown in Supplementary Table 2 . Statistical analysis Student’s t -test was applied to all statistical analyses. How to cite this article: Poh, Y.-C. et al. Generation of organized germ layers from a single mouse embryonic stem cell. Nat. Commun. 5:4000 doi: 10.1038/ncomms5000 (2014).